Predicting climate change impacts on polar bear litter size Predicting the ecological impacts of climate warming is critical for species conservation. Incorporating future warming into population models, however, is challenging because reproduction and survival cannot be measured for yet unobserved environmental conditions. In this study, we use mechanistic energy budget models and data obtainable under current conditions to predict polar bear litter size under future conditions. In western Hudson Bay, we predict climate warming-induced litter size declines that jeopardize population viability: ∼ 28% of pregnant females failed to reproduce for energetic reasons during the early 1990s, but 40–73% could fail if spring sea ice break-up occurs 1 month earlier than during the 1990s, and 55–100% if break-up occurs 2 months earlier. Simultaneously, mean litter size would decrease by 22–67% and 44–100%, respectively. The expected timeline for these declines varies with climate-model-specific sea ice predictions. Similar litter size declines may occur in over one-third of the global polar bear population. Climatic warming affects ecosystems worldwide [1] , [2] , [3] , [4] , and is a major conservation threat to Arctic species [3] , [4] , [5] . Sea ice-obligate species, such as polar bears ( Ursus maritimus ), are particularly vulnerable because their habitat is disappearing [6] , [7] , [8] , [9] , [10] . Polar bear body condition, reproduction, survival and abundance are already declining in some populations [11] , [12] , [13] , [14] , [15] , and further declines are expected with continued warming [6] , [7] , [8] , [9] , [15] , [16] . Quantifying these expectations is important for population management and conservation [10] , [16] , [17] , [18] , [19] , [20] , but predictive population models are lacking, because it is unknown how reproduction and survival will change with climatic warming [16] . These demographic parameters cannot be measured directly for climate warming scenarios, because currently observed environmental conditions differ substantially from those predicted for the future. However, future reproduction and survival may be predicted from existing data if the mechanisms causing change in these demographic parameters are known and accounted for in a mechanistic modelling framework [16] , [18] , [19] , [20] . In this study, we use mechanistic models to predict changes in litter size for pregnant females in the western Hudson Bay population under expected changes in sea ice. The mechanisms linking sea ice to litter size are well understood. For about 8 months of the year, Hudson Bay is frozen and bears hunt for seals on the sea ice [7] , [11] , [21] . Each summer, the sea ice melts and the population is forced ashore. With little to no terrestrial food available [22] , [23] , [24] , bears rely on their energy stores for survival and reproduction while on land [11] , [21] , [25] . Pregnant females enter terrestrial maternity dens in early October, where they give birth and nurse 1–3 altricial cubs until den emergence in February or March [21] , [25] , [26] . Food continues to be unavailable to females while denning, and energetic expenses of survival, gestation and lactation are met from fat and protein stores accumulated during the previous hunting season [21] , [25] . Storage energy thus limits the number of cubs that can be raised to den emergence, and the amount of storage energy available to denning females depends on the length of the previous sea ice season. Historically, polar bears came ashore in early August, but because of rising temperatures sea ice break-up has been occurring about 7–8 days earlier per decade in recent years [7] , [11] . Polar bear on-shore arrival has shifted accordingly, resulting in shortened on-ice feeding and prolonged on-shore fasting [7] , [11] . The trends towards a progressively earlier sea ice break-up and progressively earlier polar bear on-shore arrival are expected to continue with continued warming [11] , [27] , and consequent food stress is expected to lead to reduced energy stores at den entry [6] , [7] , [8] , [11] . Declines in litter size are likely because less energy is available for gestation and lactation. In this study, we derive quantitative predictions as to how future changes in sea ice break-up will affect the litter size of pregnant females. To this end, we describe the energetics of on-ice feeding, on-shore fasting and litter production in a dynamic energy budget modelling framework [28] , and evaluate how break-up date affects these energetic relationships. More specifically, our analyses proceed as follows: first, we demonstrate that litter size at den emergence can be predicted from maternal energy density at den entry (where energy density is defined as the ratio between storage energy and lean body mass [29] ; see also Supplementary Methods for definitions of all energetic terms). Next, we estimate the distribution of energy densities at den entry for females in western Hudson Bay during the early 1990s (that is, for a period before significant changes in sea ice break-up occurred [7] , [11] ), and we use this distribution to estimate their offspring production. Finally, using a dynamic energy budget model to quantify the energetic consequences of prolonged fasting and decreased feeding, we estimate how the distribution of den entry energy densities (and thus the expected distribution of litter sizes at den emergence) will change if females are forced ashore earlier in summer. 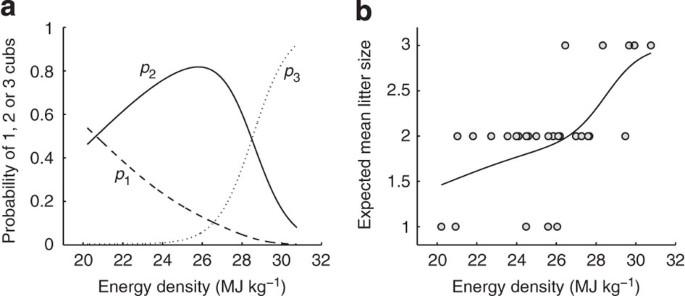Figure 1: The relationship between maternal energy density and litter size. (a) Estimated probabilities for a pregnant female polar bear to have one (p1, dashed line), two (p2, solid line) or three cubs (p3, dotted line) at den emergence as a function of maternal energy density (defined as storage energy relative to lean body mass) at den entry, as determined by multinomial logistic regression. (b) Expected mean litter size at den emergence as a function of maternal energy density at den entry (solid line), calculated asX(E/LBM)=p1(E/LBM)+2p2(E/LBM)+3p3(E/LBM). Data are observed litter sizes at den emergence as a function of maternal energy density at den entry (N=28). Relating den entry body condition to litter size We used multinomial logistic regression models [30] on data from 28 pregnant females with known litter sizes to test whether litter size at den emergence can be predicted from maternal age ( A ), storage energy [29] at den entry ( E ), energy density [29] at den entry ( E/LBM ), or certain combinations of these variables (see Table 1 and Methods for details). The model with only energy density was an excellent predictor of litter size at den emergence (likelihood ratio test, P =0.0004), and the regression probabilities of having one, two or three cubs ( Fig. 1 ) are This model also explained the data significantly better than the regression models with storage energy or age ( Table 1 ), and it was therefore used in subsequent calculations to predict litter size from body condition at den entry. Because females with insufficient energy stores do not enter maternity dens [25] , [26] , we further augmented the model by assuming an energy density threshold for reproduction [31] , [32] , setting the probability of not reproducing, p 0 , to 1 (with p 1 = p 2 = p 3 =0) if E/LBM <20.0 MJ kg −1 , and to 0 (with p 1 , p 2 and p 3 given by equations (1)–(3)) otherwise (see Methods and Supplementary Note online for details). The threshold was chosen equal to the lowest den entry energy density ever observed for a female that produced at least one cub [26] . Energy densities in our sample of females were consistent with this parameterization of the reproduction threshold, ranging from 20.2 to 30.8 MJ kg −1 at den entry. Table 1 ∣ Multinomial logistic regression models for litter size at den emergence. Full size table Figure 1: The relationship between maternal energy density and litter size. ( a ) Estimated probabilities for a pregnant female polar bear to have one ( p 1 , dashed line), two ( p 2 , solid line) or three cubs ( p 3 , dotted line) at den emergence as a function of maternal energy density (defined as storage energy relative to lean body mass) at den entry, as determined by multinomial logistic regression. ( b ) Expected mean litter size at den emergence as a function of maternal energy density at den entry (solid line), calculated as X ( E / LBM )= p 1 ( E / LBM )+2 p 2 ( E / LBM )+3 p 3 ( E / LBM ). Data are observed litter sizes at den emergence as a function of maternal energy density at den entry ( N= 28). Full size image Predicted changes in litter size with earlier ice break-up Next, we followed a two-step approach to determine how the distribution of energy densities at den entry, and thus the distribution of litter sizes at den emergence, will be affected if pregnant females are forced ashore early (see Methods for details). First, we determined the distribution of energy densities at on-shore arrival and den entry in a representative sample of adult females without dependent offspring ( N= 40) caught during the early 1990s. Second, using a dynamic energy budget model [28] , [31] , [32] to track changes in body mass, storage energy and energy density due to feeding, somatic maintenance and movement, we estimated how energy densities at on-shore arrival and den entry, and thus litter sizes at den emergence, will change with earlier on-shore arrival (see Fig. 2 and Methods). This second step requires on-ice feeding rate estimates to quantify the energetic impacts of a shortened hunting period. However, on-ice feeding rates are unknown for Hudson Bay, and it is also unclear how these rates vary seasonally. We therefore considered two feeding scenarios, 'Early Feeding' and 'Late Feeding', which estimate likely boundaries for the impacts of earlier on-shore arrival ( Fig. 2 ). Early Feeding assumes that bears can only accumulate storage energy until the end of May (that is, during, and shortly after, seal pupping [33] , [34] , [35] ) and that feeding during the remaining on-ice period is reduced to rates that are just sufficient for bears to maintain acquired body mass. For earlier on-shore arrival, the Early Feeding scenario probably overestimates litter sizes at den emergence, because it only considers prolonged fasting but not potential losses in feeding. In the Late Feeding scenario, we account for both the prolonged fast and for missed feeding opportunities by assuming high energy intake during June and July, similar to intake rates in the High Arctic [35] . Bears accumulate much of their storage energy just before on-shore arrival with Late Feeding, so that females forced ashore early not only fast longer before den entry but they also come ashore in poorer body condition. This scenario probably overestimates the energetic impact of earlier on-shore arrival (thus underestimating litter sizes at den emergence), because summer feeding rates in Hudson Bay are likely lower than in the High Arctic ( Supplementary Methods ). 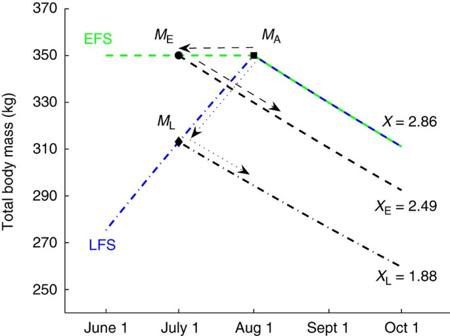Figure 2: Method to estimate changes in litter size under earlier on-shore arrival. The logic of our analyses is illustrated for a female with straight-line body lengthL=1.9 m that hunted on the sea ice until 1 August and came ashore with body massMA=350 kg on that date (solid square). We first establish her body masses before and after on-shore arrival, subject to the constraintMA=350 kg. Before on-shore arrival body masses (1 June to 1 August) are estimated by projectingMAbackwards in time under the Early (green dashed line, EFS) and Late Feeding (blue dot-dashed line, LFS) scenarios, respectively. After 1 August, body mass is lost because of on-shore fasting in both scenarios (green-blue dashed line), resulting in a den entry (1 October) body mass of 311.1 kg. Energy density at den entry is thus 30.25 MJ kg−1, implying an expected mean litter sizeX=2.86 (equations (1)–(3)). Next, on-shore fasting is initiated at an earlier date (1 July in this example; arrows) with on-shore arrival body mass equalling the body mass obtained for that date under Early and Late Feeding,MEandML, respectively. In this example,ME=350 kg (solid circle) andML=313.1 kg (solid diamond). Mass loss due to fasting then results in den entry body masses 292.4 kg and 259.6 kg, den entry energy densities 28.64 MJ kg−1, and 25.50 MJ kg−1, and expected mean litter sizesXE=2.49 andXL=1.88, under the Early (dashed line) and Late (dot-dashed line) Feeding scenarios, respectively. Figure 2: Method to estimate changes in litter size under earlier on-shore arrival. The logic of our analyses is illustrated for a female with straight-line body length L =1.9 m that hunted on the sea ice until 1 August and came ashore with body mass M A =350 kg on that date (solid square). We first establish her body masses before and after on-shore arrival, subject to the constraint M A =350 kg. Before on-shore arrival body masses (1 June to 1 August) are estimated by projecting M A backwards in time under the Early (green dashed line, EFS) and Late Feeding (blue dot-dashed line, LFS) scenarios, respectively. After 1 August, body mass is lost because of on-shore fasting in both scenarios (green-blue dashed line), resulting in a den entry (1 October) body mass of 311.1 kg. Energy density at den entry is thus 30.25 MJ kg −1 , implying an expected mean litter size X =2.86 (equations (1)–(3)). Next, on-shore fasting is initiated at an earlier date (1 July in this example; arrows) with on-shore arrival body mass equalling the body mass obtained for that date under Early and Late Feeding, M E and M L , respectively. In this example, M E =350 kg (solid circle) and M L =313.1 kg (solid diamond). Mass loss due to fasting then results in den entry body masses 292.4 kg and 259.6 kg, den entry energy densities 28.64 MJ kg −1 , and 25.50 MJ kg −1 , and expected mean litter sizes X E =2.49 and X L =1.88, under the Early (dashed line) and Late (dot-dashed line) Feeding scenarios, respectively. Full size image During the early 1990s, the energy density distribution of adult females without dependent offspring ranged from 13.8 to 31.4 MJ kg −1 (mean: 25.7±0.67 MJ kg −1 ) at mean on-shore arrival (1 August) and from 9.2 to 28.3 MJ kg −1 (mean: 22.2±0.72 MJ kg −1 ) at den entry (1 October). The proportions of females producing zero, one, two or three cubs were estimated as p 0 =0.275, p 1 =0.155, p 2 =0.517 and p 3 =0.053 using the regression model described above. Expected mean litter size, including females with zero cubs, was therefore X =1.35 (95% confidence interval (CI): 1.08–1.62). Expected mean litter size conditional on producing at least one cub was X *=1.86 (95% CI: 1.77–1.94), which closely matches the observed value of 1.84 during 1980–1992 [36] , suggesting that our sample is representative. With earlier on-shore arrival, substantial declines in mean litter size ( X ) are predicted for both feeding scenarios ( Fig. 3 ). With Early Feeding, we predict X =1.05 if bears come ashore on 1 July and X =0.75 for on-shore arrival on 1 June. Predicted declines are stronger with Late Feeding, with X =0.45 for on-shore arrival on 1 July and no reproduction ( X =0) for on-shore arrival before 7 June. For both scenarios, we predict the proportions of females with twins and triplets to decline monotonically and the proportion of non-reproducing females to increase monotonically ( Fig. 3a,b ). Declines in twin and triplet production will precede declines in the proportion of females having singletons, because some females will move from having twins to having singletons, whereas others will move from having singletons to not reproducing. These predicted changes are consistent with patterns already observed in western Hudson Bay where females are now forced ashore 1–2 weeks earlier than during the early 1990s, and both body condition and reproduction have declined [7] , [11] . More precise data suitable for model validation do not exist, and it is noteworthy in this regard that the predicted litter size changes will be difficult to document if monitoring focuses on X * rather than on X ( Fig. 3c,d ). 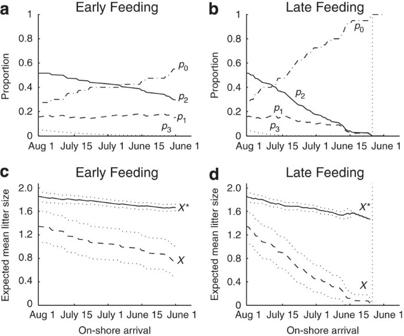Figure 3: Predicted changes in litter size as a function of on-shore arrival date. (a,b) Expected proportions of pregnant female polar bears in western Hudson Bay to produce zero (p0, dot-dashed line), one (p1, dashed line), two (p2, solid line) and three (p3, dotted line) cubs as a function of on-shore arrival date under the Early and Late Feeding scenarios, respectively. (c,d) Expected mean litter size (X, dashed line) and expected mean litter size conditional on producing at least one cub (X*, solid line) as a function of on-shore arrival date under Early and Late Feeding, respectively. Dotted lines show 95% confidence intervals. The vertical dotted lines inbanddmark 7 June, the on-shore arrival date before which reproduction becomes impossible with Late Feeding. Figure 3: Predicted changes in litter size as a function of on-shore arrival date. ( a , b ) Expected proportions of pregnant female polar bears in western Hudson Bay to produce zero ( p 0 , dot-dashed line), one ( p 1 , dashed line), two ( p 2 , solid line) and three ( p 3 , dotted line) cubs as a function of on-shore arrival date under the Early and Late Feeding scenarios, respectively. ( c , d ) Expected mean litter size ( X , dashed line) and expected mean litter size conditional on producing at least one cub ( X *, solid line) as a function of on-shore arrival date under Early and Late Feeding, respectively. Dotted lines show 95% confidence intervals. The vertical dotted lines in b and d mark 7 June, the on-shore arrival date before which reproduction becomes impossible with Late Feeding. Full size image Correctly predicting the population-level impacts of climate change is a challenge in many species because the data required to parameterize population models for climate change scenarios usually cannot be obtained before environmental changes occur [16] , [18] , [19] , [20] . We therefore advocate models that explicitly consider the mechanisms by which environmental variables affect individuals and populations [16] , [18] , and especially dynamic energy budget models, as tools to predict vital rates and other population dynamics determinants (for example, density dependence [32] ) for yet-to-be-observed conditions. Although the results of this study are specific to polar bears, the approach itself is broadly applicable to other species [16] , [18] . Energy budget models have, for example, been used to study the energetic consequences of climate-associated mismatches between reproductive timing and resource availability in birds [37] . In mammals, energy budget models have been applied to predict distribution changes in bats under climate warming [38] . However, detailed mammalian models that mechanistically link climate change to individual energetics and consequent changes in vital rates are new [18] , and our analyses provide the first mechanistic prediction for changes in polar bear reproduction under climate warming. The approach synthesizes long-term research on polar bear physiology, ecology and behaviour in a common modelling framework that only requires data obtainable under current conditions. Thus, we were able to overcome the absence of data specifying the empirical relationship between polar bear litter size and future environmental conditions, and our predictions are the logical consequence of the current knowledge on this species. The next logical step is to connect the ecological model presented here (predicting litter size as a function of on-shore arrival date) with climate and sea ice models (predicting future break-up, and thus [11] polar bear on-shore arrival dates) to obtain predictions for the timeframe within which litter size declines are to be expected. We illustrate this process using the sea ice model of Joly et al . [27] , which was developed specifically for the Hudson Bay region. Assuming the Intergovernmental Panel on Climate Change Special Report on Emissions Scenarios A2 scenario [39] , their model suggests that break-up date in western Hudson Bay could occur in early- to mid-June by around mid-century [27] , which, in turn, would imply a shift in polar bear on-shore arrival to about 1 July [11] (that is, to about 1 month earlier than during the 1990s). For this case, our model predicts that 40–73% of pregnant females will be unable to produce a litter (compared with ∼ 28% during the early 1990s), where the lower and upper bounds are given by the Early and Late Feeding scenarios, respectively ( Fig. 3a,b ). Simultaneously, the proportions of females producing one, two and three cubs will decline to 16, 43 and 1% with Early Feeding ( Fig. 3a ), and to 10, 18 and 0% with Late Feeding ( Fig. 3b ), respectively (compared with an estimated 16, 52 and 5% during the early 1990s; see Results ). In sum, mean litter size would decline to somewhere between X =0.45 (Late Feeding) and X =1.05 (Early Feeding) by mid-century ( Fig. 3c,d ), a relative decline of 22–67% compared with the early 1990s when X =1.35. These predictions are probably conservative (that is, the actual declines in litter size under the sea ice scenario of Joly et al . [27] may be larger than outlined here) because we have not considered carry-over effects of low female body condition between consecutive years of low sea ice [7] (see Methods). The timeline for litter size changes discussed in the previous paragraph is specific to the sea ice projections of Joly et al . [27] Other climate and sea ice models could be connected to our litter size model in a similar manner, and such analyses might yield slower or faster litter size declines than discussed above. However, although the predicted rate of decline may be affected by the choice of climate and sea ice model, litter size declines will occur under any warming scenario that causes earlier sea ice break-up ( Fig. 3 ), and such a shortening of the sea ice season is consistently predicted by climate-linked sea ice models [39] . Our model predictions rest on the parsimonious assumption that all ecological dynamics, except on-shore arrival date, remain unchanged (see Methods). Furthermore, wherever possible, we made model assumptions that would yield conservative predictions of litter size (for example, strong homeostasis, no increase in energy expenditure towards den location, excavation and maintenance under future environmental conditions, and no changes in thermoregulation while denning; see Supplementary Methods for details). However, certain shifts in behaviour, reproductive strategy or ecosystem processes could be hypothesized to alleviate some of the expected food stress on polar bears, thereby slowing the predicted litter size declines to some extent, and it is worth considering whether and how such changes might affect our litter size predictions. For example, it has been speculated that polar bears could compensate for losses in on-ice feeding by using terrestrial food sources [40] . However, such a strategy is unlikely to ameliorate the predicted impacts of earlier on-shore arrival because food sources that could provide significant storage energy are unavailable on land [22] , [23] , [24] . Alternatively, polar bears could avoid a prolonged pre-denning fast (and consequent reductions in litter size) if blastocyst implantation and maternity den entry occurred earlier under earlier sea ice break-up (in our analyses, we assumed that den entry always occurs on 1 October, irrespective of on-shore arrival date). Whether such changes in denning phenology are physiologically possible is unknown, but this is unlikely if implantation has evolved to photoperiod as the environmental cue [41] . However, even if polar bears could adjust to earlier denning, we consider it unlikely that such an adjustment would counteract the predicted litter size declines. Current den entry is timed such that den emergence and the following return to sea ice align with the period when seals are most available (for example, during pupping) [21] . With earlier den entry and parturition, den emergence would also occur earlier, thus creating a potential mismatch between food requirements of newly emerged family groups and peak food availability. The ability of females to replenish their energy stores to sustain lactation after den emergence could be compromised in this case, so that a potential gain in litter size achieved by earlier den entry might be negated by increased cub mortality after den emergence. Such negative impacts of a climate-induced mismatch between reproductive timing and resource availability have been documented, for example, for caribou ( Rangifer tarandus ) offspring survival [42] . Another way to counteract poor body condition at den entry, and thus avoid or slow down litter size declines, may be for females to skip reproduction for one or more consecutive years in cases where reduced energy stores would lead to reduced litter size. Non-reproducing females could return onto the sea ice at freeze-up (November–December) [7] , [11] to feed for an additional year and possibly increase their storage energy before re-attempting reproduction. In this study, we cannot evaluate whether individuals could gradually increase their body condition by skipping reproduction, and whether this would significantly affect the predicted distributions of den entry energy density and litter size, because insufficient data on on-ice feeding prevented modelling between-year carry-over effects of storage energy. However, we believe that explicitly accounting for skipped reproduction would not result in significantly slower litter size declines than predicted here: first, our sample distribution of den entry energy densities probably already accounts for the effects of skipped reproduction in a proportion of females, because an estimated 28% of females did not den during the early 1990s ( Fig. 3a,b ). Second, although an increasing proportion of females could skip reproduction with earlier ice break-up ( Fig. 3a,b ), it would also become more difficult for non-reproducing females to increase their storage energy until the following fall with climate warming, because not only the break-up of sea ice would be earlier but fall freeze-up would also be delayed, possibly by as much as 3–4 weeks [27] . The storage energy saved by not reproducing would thus be partially lost again with the extended fasting season, and non-reproducing individuals would still have fewer opportunities to accumulate new storage energy in spring. Furthermore, even if individuals could avoid a decrease in litter size by skipping reproduction, their lifetime reproductive output, and thus population growth rate, would still decrease with reduced sea ice, because the potential gain in litter size comes at the expense of an increased inter-birth interval. Full evaluation of the energetic and reproductive consequences of potential shifts in denning phenology or of shifts in inter-birth interval requires a dynamic energy budget model that incorporates the entire reproductive cycle of polar bears. Such a model could also be used to understand and predict the impacts of reduced sea ice on other components of reproduction, including lactation, cub growth, cub survival to independence, and age at first reproduction [16] . Each of these components depends, where at least partially on storage energy and could thus be negatively affected by sea ice reductions and associated reductions in feeding. Low storage energy, for instance, may result in low milk production, which may slow cub growth and/or increase cub mortality [43] , [44] . Slower cub growth, in turn, may result in delayed sexual maturity and age at first reproduction [46] . The present model could be extended to include these life history traits as new data on polar bear physiology and feeding ecology become available. Data requirements for such a more comprehensive model have been discussed eflsewhere [16] . Our analyses, however, further emphasize the need to quantify current on-ice feeding rates. Declining feeding opportunities (and resultant declines in body condition, reproduction and survival) constitute the biggest concern for polar bears under climatic warming [6] , [8] , [16] , and dynamic energy budget models have the potential to predict body condition, reproduction and survival under yet-to-be-observed feeding conditions [16] , [28] , [45] , [47] . We therefore expect this modelling approach to advance our ability to understand and predict the impacts of climate warming on polar bear populations. However, to model how reduced energy intake would affect polar bear reproduction and survival, it is imperative to first understand energy intake under current and past conditions. For example, with better information on on-ice feeding rates, our model could be improved to not only estimate boundaries for the energetic impacts of earlier on-shore arrival ( Figs 2 and 3 ) but to also determine the most likely trajectory for future litter size declines. The litter size predictions provided in this study serve as another indicator that the western Hudson Bay population will probably not remain viable under predicted climatic conditions. Body condition, reproduction, survival and abundance have already declined in this population [11] , [12] , and our analyses indicate that further substantial declines in litter size are likely under expected sea ice loss, even in the conservative Early Feeding scenario. These declines will probably be accompanied by declines in survival and other reproductive components, because these parameters are also limited by storage energy [16] . Outside western Hudson Bay, over one-third of the global polar bear population follows similar patterns of seasonal on-ice feeding and on-shore fasting [7] , [9] . The physiological arguments put forth in our study also suggest future litter size declines in these populations, although the rates of decline may differ from the western Hudson Bay population and must be evaluated separately to account for population-specific sea ice changes. Relating den entry body condition to litter size Pregnant female polar bears ( N= 28; ages: 5.8–20.8 years) were captured on shore from August to October (1980–1992) in the western Hudson Bay denning area. Age ( A ), straight-line body length ( L ) and axillary girth ( G ) were recorded for each bear using standard procedures [48] . For sampling details and capture procedures see ref. 49 where these data were previously reported in a different context. None of these bears were weighed, so we estimated body masses ( M ) using the morphometric equation [50] M = e −9.03 L 1.29 G 1.60 . We assumed den entry on 1 October [26] and used the mass loss curve for fasting, resting, non-growing and non-reproducing polar bears in a thermoneutral state [29] to scale body masses to this date. From body mass on 1 October and straight-line body length, we estimated storage energy at den entry ( E ) and energy density at den entry ( E/LBM ) for each female using the body composition model of ref. 29 . All females were recaptured the following spring at den emergence (late-February to late-March) when litter sizes were recorded [49] . We used multinomial logistic regression models [30] to test whether litter size at den emergence can be predicted from maternal age, storage energy at den entry, energy density at den entry, or certain combinations of these variables ( Table 1 ). Storage energy, commonly used in dynamic energy budget modelling as a predictor variable for reproductive output [28] , [31] and necessary for den survival, gestation and lactation [25] , was a priori considered a likely determinant for litter size. However, we also hypothesized that energy density may predict litter size better than storage energy alone because energy density explicitly relates available storage energy to the energetic requirements of maternal somatic maintenance (that is, survival) while denning [29] . In addition, we considered regression models containing the covariate age, either by itself or in combination with storage energy or energy density, because age has been previously suggested to influence reproductive success in polar bears [21] , [49] . Thus, we fitted a total of five multinomial logistic regression models to the litter size data ( Table 1 ), determining the probabilities of having one, two or three cubs, p 1 , p 2 and p 3 , as a function of the respective model covariates. We used likelihood ratio tests to determine covariate significance in each model, and Akaike's Information Criterion adjusted for small sample size [51] , AIC c , for model selection. Energy density was an excellent predictor of litter size (likelihood ratio test, P =0.0004), and the model with energy density as the only covariate (equations (1)–(3)) explained the data significantly better than all other models ( Table 1 ). In subsequent calculations, we therefore used the regression model with only energy density to predict litter size. Data on non-reproducing females were unavailable because females with insufficient energy stores for denning survival, gestation and lactation do not enter maternity dens [25] , [26] . Thus, we could not determine the probability of not reproducing, p 0 , by regression. Instead, we augmented the regression model by assuming a threshold for reproduction [31] , [32] : mature females produce at least one cub if their energy density is above the threshold at den entry, whereas below the threshold they cannot reproduce. The chosen threshold was 20.0 MJ kg −1 , the lowest den entry energy density ever observed for a female that produced at least one cub [26] . Formally, we set p 0 ( E/LBM )=1 (and p 1 = p 2 = p 3 =0), if E/LBM <20.0 MJ kg −1 on 1 October, and p 0 ( E/LBM )=0 (and p 1 , p 2 , p 3 given by equations (1)–(3)) otherwise. The simplifying assumption of such a reproduction threshold is supported by dynamic energy budget theory [52] and has also been applied in other mammalian dynamic energy budget models [31] , [32] . Our parameterization of this threshold likely provides a conservative assessment of future litter size. Potential deviations from this threshold would not affect our qualitative conclusions and are unlikely to substantially alter numerical predictions of future litter size ( Supplementary Note, Supplementary Figs. S1, S2 ). Predicted changes in litter size with earlier ice break-up Next, we determined how the distribution of energy densities at den entry, and thus the distribution of litter sizes at den emergence, will be affected if pregnant females are forced ashore earlier because of earlier sea ice break-up. First, we determined the distribution of on-shore arrival body masses during the early 1990s, using adult females without dependent offspring caught non-selectively in the western Hudson Bay denning area during the summer fasting periods of 1989–1996 ( N= 40; ages: 4.8–22.8 years). All bears were weighed, and straight-line body lengths and ages were determined as above. Body masses were scaled (using the mass loss curve of ref. 29 ) from capture date to 1 August, the mean on-shore arrival date in 1991–1998 [11] . In subsequent calculations, we denote body mass for a given female on 1 August as M A , and we write t 0 for the reference on-shore arrival date of 1 August. Next, we considered how on-shore arrival body masses will differ if females are forced ashore t days before t 0 . We assumed that mass gain until on-shore arrival always follows the mass gain curve during the early 1990s, irrespective of arrival date (that is, we assumed all ecological dynamics except arrival date unchanged, and in particular we assumed no carry-over effects of body mass between consecutive years). Estimating the impacts of earlier on-shore arrival on the distribution of on-shore arrival body masses then amounts to estimating M ( t 0 −t ) for each female (that is, realized body mass t days before 1 August) subject to the constraint that her body mass on 1 August was M ( t 0 )= M A ( Fig. 2 ). Direct estimates of M ( t 0 −t ) from body mass time series were impossible because bears are not sampled on sea ice in this population. Instead, we estimated M ( t 0 −t ) for each female by projecting body masses backwards in time from M ( t 0 )= M A . Such projections require on-ice feeding rate estimates, but feeding rates are unknown for Hudson Bay and it is unclear when bears accumulate most of their storage energy. Hence, we considered two feeding scenarios, termed 'Early Feeding' and 'Late Feeding'. In Early Feeding, we assumed that bears may accumulate storage energy until the end of May and that energy intake during the remaining on-ice period is lower and just sufficient to maintain acquired body mass. In this case, earlier on-shore arrival results in prolonged fasting but not in poorer body condition when coming ashore. In Late Feeding, we accounted for the possibility that energy intake might be high during June and July, comparable with intake rates in the High Arctic [35] . In this case, bears accumulate most of their storage energy just before on-shore arrival, so that females forced ashore early not only fast longer before den entry but they also come ashore in poorer body condition. Formalizing the above assumptions as follows, we estimated M ( t 0 −t ) for each female on all dates from 1 June to 1 August ( t =0,...,61), writing M ( t 0 −t )≡ M E ( t 0 −t ) and M ( t 0 −t )≡ M L ( t 0 −t ) for the Early and Late Feeding scenarios, respectively. For Early Feeding, body mass t days before 1 August equals body mass on 1 August, so that M E ( t 0 −t )= M A for t =0,...,61. With Late Feeding, storage energy is accumulated until 1 August, so that M L ( t 0 −t )< M A for t >0. To estimate M L ( t 0 −t ), we assumed feeding rates as in the High Arctic [35] and used the following dynamic energy budget model to calculate body mass changes backwards in time from the initial condition M ( t 0 )= M A : The model tracks changes in storage energy (and thus also changes in body mass and energy density [29] ) over time due to feeding, somatic maintenance and movement, and is formally derived in Supplementary Methods . A summary of parameter definitions and estimates is provided in Table 2 . Table 2 ∣ Model parameters for the dynamic energy budget model of adult female polar bears without dependent offspring (equation (4)). Full size table For each feeding scenario and each on-shore arrival date t 0 − t , we then used the distribution of body masses M ( t 0 − t ) as initial conditions for a fasting season initiated t days before 1 August. Assuming that den entry always occurs on 1 October, irrespective of on-shore arrival date, we obtained the distribution of den entry body masses by projecting M ( t 0 − t ) forwards in time to 1 October for each female, again using the mass loss curve of ref. 29 . The distribution of den entry energy densities was then estimated from straight-line body lengths and den entry body masses [29] , and the probabilities of producing zero, one, two or three cubs were estimated for each female from the regression model described above. Summing these probabilities over all females and normalizing by sample size yielded the expected proportions of females producing zero, one, two or three cubs, given on-shore arrival date and feeding scenario. From these proportions, we also calculated expected mean litter size ( X ) and expected mean litter size conditional on producing at least one cub ( X *) as a function of on-shore arrival date and feeding scenario. The logic of these calculations is illustrated in Figure 2 . Data sources and statistical analyses The denning data used to derive regression equations (1)–(3) were previously reported in ref. 49 , and these data were collected and made available by Environment Canada. The body condition data on adult females without dependent offspring, used to determine the distribution of on-shore arrival body masses during the early 1990s, were collected by M. Ramsay of the University of Saskatchewan during non-selective sampling of the western Hudson Bay population. The two data sets were collected independently from each other and do not overlap. Statistical results were considered significant at P ≤ 0.05. Means are presented as ±1 standard error of the mean. How to cite this article: Molnár, P.K. et al . Predicting climate change impacts on polar bear litter size. Nat. Commun. 2:186 doi: 10.1038/ncomms1183 (2011).